Long-living terahertz magnons in ultrathin metallic ferromagnets The main idea behind magnonics is to use the elementary magnetic excitations (magnons) for information transfer and processing. One of the main challenges, hindering the application of ultrafast terahertz magnons in magnonics, has been the short lifetime of these excitations in metallic ferromagnets. Here, we demonstrate that the engineering of the electronic structure of a ferromagnetic metal, by reducing its dimensionality and changing its chemical composition, opens a possibility to strongly suppress the relaxation channels of terahertz magnons and thereby enhance the magnons’ lifetime. For the first time, we report on the long-lived terahertz magnons excited in ultrathin metallic alloy films. On the basis of the first-principles calculations, we explain the microscopic nature of the long lifetime being a consequence of the peculiar electronic hybridizations of the species. We further demonstrate a way of tailoring magnon energies (frequencies) by varying the chemical composition of the film. Spintronics takes advantage of the electron’s spin as an information carrier. This has already opened totally new opportunities for information processing by involving spin-dependent phenomena in solids [1] . The elementary magnetic excitations (magnons) can also be used to carry information [2] , [3] , [4] . In the quickly developing field of magnonics, the aim is to use the magnons for information transfer and processing [2] , [3] , [4] . When a magnon propagates through a magnetic medium, no electrical charge transport is involved and hence no electrical losses, creating Joule heating, take place. This is the fundamental advantage of using magnons as information carriers. In addition to that, magnons cover a very wide frequency window, from gigahertz up to a few hundreds of terahertz. They possess a lifetime ranging from a few tenths of a microsecond down to tens of femtoseconds, depending on the frequency. The excitation energy and the lifetime have an important impact on the performance of magnon-based devices. Since the magnon dispersion relation in ferromagnets is parabolic in the first approximation, the larger the excitation frequency, the faster are the magnons. This means that the use of high-frequency (terahertz) magnons would provide a great opportunity for the design of ultrafast devices. However, one of the main challenges for using terahertz magnons is their short lifetime in metallic ferromagnets [5] , [6] , [7] , [8] , [9] , [10] , [11] , [12] , [13] , [14] , [15] , [16] . Hence, the discovery of a low-damping material would push the progress in the field of terahertz magnonics one big step further. The strong damping of terahertz magnons in itinerant ferromagnets arises mainly due to the presence of single-particle excitations (known as Stoner excitations) in the same energy window as the magnons. As a result, the terahertz magnons in metallic ferromagnets feature a very short lifetime, only up to a few tens of femtoseconds [5] , [11] , [12] , [13] , [14] , [17] . The decay of magnons into Stoner excitations is usually referred to as Landau damping. There are other sources of damping, for example, phonon and impurity scattering, two-magnon scattering and spin–orbit damping. These damping mechanisms are not as strong as Landau damping and are only important for the limit of low-frequency (gigahertz) excitations [18] . If there are no low-energy Stoner excitations, with energies in the range of magnons’ energy, the Landau damping will be inoperative and magnons shall live for a longer time. In principle, in ferro(i)magnetic insulators, for example, yttrium iron garnet [19] , or half metals, for example, Heusler alloys [8] , [9] , [15] , the low-energy Stoner excitations are not allowed (in insulators, the density of states of both spin-up and spin-down electrons near the Fermi level is zero; and in half metals, the density of states of one spin character near the Fermi level is zero). Therefore, one expects that the Landau damping is not operative and hence terahertz magnons shall exhibit a long lifetime. However, very little is known about the terahertz magnons and their lifetime in these materials. In addition, the structural complexity and the extreme difficulty of preparing high-quality samples in the form of thin films and nano-structured devices would hinder, to a large extent, their potential applications in terahertz magnonics. One of the disadvantages of magnetic insulators is that they are usually very hard and are not compatible with nano-fabrication using conventional lithographic methods (for terahertz magnonics, the size of the devices shall be on the order of the propagation distance of these magnons, that is, a few nanometres). One of the disadvantages of Heusler alloys is that the structural disorder and anti-site defects strongly suppress their half-metallic character, which is responsible for the low magnon damping in these materials [20] . Here, we report on an alternative material, an ultrathin film of iron–palladium (Fe–Pd) alloy, with a low Landau damping for the potential application in terahertz magnonics. The Landau damping parameter of this system is comparable to the one of the ferromagnetic insulators. On the basis of our results of the frequency and wave vector-resolved measurements of the magnons’ lifetime, we show that the lifetime of magnons is rather long in this system. We further demonstrate that the excitation frequencies can be tuned by changing the Fe content in the sample. Probing magnons in FePd alloy films on Pd(001) An ultrathin FePd alloy film with a thickness of two atomic layers was grown on a Pd(001) surface. The film was prepared using the so-called mild annealing technique of Fe monolayer on the Pd(001) surface. A structurally well-ordered face-centered tetragonal alloy film was obtained. The film is chemically disordered [21] . Spin-polarized high-resolution electron energy loss spectroscopy (SPEELS) was used to study the magnetic excitations. Due to its monolayer sensitivity, possibility of measuring magnetic excitations over the whole surface Brillouin zone and the capability of investigating spin-dependent scattering, SPEELS is a powerful technique for probing terahertz magnons in ultrathin ferromagnetic films [22] , [23] , [24] , [25] , [26] , [27] , [28] , [29] , [30] . A schematic representation of the scattering geometry in our SPEELS experiments is shown in Fig. 1a . Typical SPEELS spectra recorded at an incident electron energy of 6 eV and at a wave vector of q =0.6 Å −1 are presented in Fig. 1b . The spectra are recorded on a two-atomic-layer-thick FePd film. I ↓ ( I ↑ ) denotes the intensity of the scattered beam when the spin polarization of the incident electrons is parallel (antiparallel) to the macroscopic magnetization. The SPEELS spectra are dominated by a peak located at zero energy loss. This peak is the so-called quasi-elastic peak and is caused by the electrons that are quasi-elastically scattered (electrons with the energy loss of zero during the scattering process). These electrons do not contribute to inelastic excitations. A well-defined excitation peak appears at ~50 meV in the I ↓ spectrum. Due to the conservation law of the total angular momentum, the magnons are only excited by incidence of minority electrons ( S =−1/2 ħ , spin polarization parallel to the sample magnetization). The difference spectrum, defined as I ↓ − I ↑ , is represented by the green solid circles, showing a well symmetric shape. To reduce the influence of nonmagnetic excitations, such as vibrational excitations, the difference spectrum was used for further data analysis. The spectra were measured for different wave vectors and along the main symmetry axes of the surface Brillouin zone. 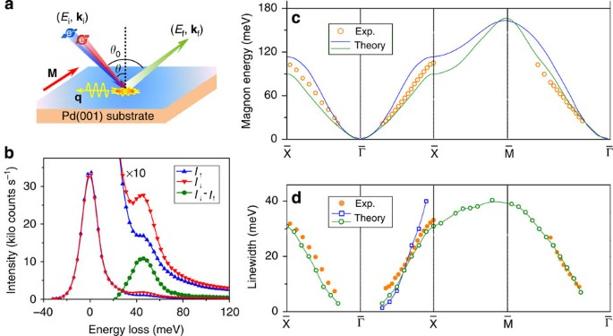Figure 1: The magnon dispersion relation and linewidth. (a) A schematic representation of the scattering geometry in our SPEELS experiments.Mis the magnetization,Ei(Ef) is the energy of the incident (scattered) beam,ki(kf) is the wave vector of the incident (scattered) beam,θis the incident angle, andθ0=80° is the angle between the incident beam and the scattered beam.qis the wave vector of the excited magnon. (b) Typical SPEELS spectra at the wave vector of 0.6 Å−1, recorded on a two-atomic-layer-thick FePd alloy film on Pd(001) atT=13 K. The red (I↓) and blue (I↑) spectra represent the intensity of the scattered electrons for the spin polarization of the incident beam parallel and antiparallel to macroscopic magnetization, respectively. To clearly see the magnon excitation peak,I↓,I↑and the difference spectra (I↓–I↑) in the region of positive energy loss are multiplied by a factor of 10 and are shown in the same graph. The difference spectrum (I↓–I↑) is represented by green solid circles. The peak at about 50 meV in the spectra is due to the magnon excitations. (c) The experimental (exp.) and theoretical magnon dispersion relation along theanddirections. The length ofis 1.15 Å−1, and the length ofis 1.61 Å−1. The empty circles represent the experimental results. The blue and green solid curves denote the magnon dispersion relation of a two-atomic-layer-thick Fe50Pd50alloy film on Pd(001) and one atomic layer of Fe film on Pd(001), respectively. (d) The intrinsic magnon linewidth alonganddirections. The solid circles denote the experimental results. The open squares and circles represent the calculated results of a two-atomic-layer-thick Fe50Pd50alloy film on Pd(001) and one atomic layer of Fe film on Pd(001), respectively. Figure 1: The magnon dispersion relation and linewidth. ( a ) A schematic representation of the scattering geometry in our SPEELS experiments. M is the magnetization, E i ( E f ) is the energy of the incident (scattered) beam, k i ( k f ) is the wave vector of the incident (scattered) beam, θ is the incident angle, and θ 0 =80° is the angle between the incident beam and the scattered beam. q is the wave vector of the excited magnon. ( b ) Typical SPEELS spectra at the wave vector of 0.6 Å −1 , recorded on a two-atomic-layer-thick FePd alloy film on Pd(001) at T =13 K. The red ( I ↓ ) and blue ( I ↑ ) spectra represent the intensity of the scattered electrons for the spin polarization of the incident beam parallel and antiparallel to macroscopic magnetization, respectively. To clearly see the magnon excitation peak, I ↓ , I ↑ and the difference spectra ( I ↓ – I ↑ ) in the region of positive energy loss are multiplied by a factor of 10 and are shown in the same graph. The difference spectrum ( I ↓ – I ↑ ) is represented by green solid circles. The peak at about 50 meV in the spectra is due to the magnon excitations. ( c ) The experimental (exp.) and theoretical magnon dispersion relation along the and directions. The length of is 1.15 Å −1 , and the length of is 1.61 Å −1 . The empty circles represent the experimental results. The blue and green solid curves denote the magnon dispersion relation of a two-atomic-layer-thick Fe 50 Pd 50 alloy film on Pd(001) and one atomic layer of Fe film on Pd(001), respectively. ( d ) The intrinsic magnon linewidth along and directions. The solid circles denote the experimental results. The open squares and circles represent the calculated results of a two-atomic-layer-thick Fe 50 Pd 50 alloy film on Pd(001) and one atomic layer of Fe film on Pd(001), respectively. Full size image Magnon dispersion relation and lifetime To extract the excitation energy and lifetime, the difference spectra were fitted using a convolution of a Gaussian and a Lorentzian function, in which the Gaussian represents the instrumental broadening and the Lorentzian represents the intrinsic lifetime broadening [13] , [14] . For a detailed description of the fitting procedure, see Supplementary Note 1 and Supplementary Figure 1 . The results of the data analysis are presented in Fig. 1c,d . Taking the in-plane lattice constant of the alloy film, the same as the one of the Pd substrate (3.89 Å), the length of the direction is 1.15 Å −1 , and the length of is 1.61 Å −1 . The magnon dispersion relation is shown in Fig. 1c . The magnon energy shows a clear dependence on the wave vector and reaches a value of 105 meV at the point. Figure 1d shows the intrinsic linewidth of the magnon excitation peak as a function of the wave vector. At the -point, the wave vector of 1.15 Å −1 , the linewidth is only 30 meV, which is smaller than the value observed for other metallic ferromagnets [13] , [14] , [29] , [31] , [32] . The lifetime of excitations can simply be obtained using the expression: τ =2 ħ /Δ ε , where ħ is reduced Planck constant and Δ ε is intrinsic linewidth, shown in Fig. 1d . The data of such analysis are presented by solid squares in Fig. 2a . Comparing this data to the corresponding data of a two-atomic-layer-thick Fe film on W(110), one clearly observes that the lifetime in the FePd film is longer (see Fig. 2b ). Note that the long lifetime is especially important for the high-energy magnons (the magnons with a large wave vector), since these magnons exhibit high group and phase velocities and are favoured for ultrafast information transfer. 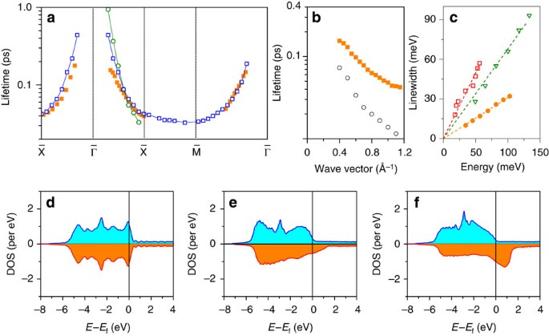Figure 2: The magnon lifetime and spin-resolved density of states. (a) The magnon lifetime as a function of the wave vector. Solid squares represent the measured magnon lifetime of a two-atomic-layer-thick FePd alloy film on Pd(001) atT=13 K. The open squares and circles denote the calculated magnon lifetime for a two-atomic-layer-thick Fe50Pd50alloy film on Pd(001) and one atomic layer of Fe film on Pd(001), respectively. (b) The experimental magnon lifetime of the FePd alloy film (solid squares) compared with the one of a two-atomic-layer-thick Fe film on W(110) (empty circles). (c) The magnon linewidth as a function of the magnon energy. The results of the FePd alloy film on Pd(001) (solid circles) are compared with the ones of one atomic layer of Fe on W(110) (empty squares) and two atomic layers of Fe on W(110) (empty triangles). The dashed lines represent linear fits to the experimental data. (d) Density of states (DOS) of Pd atoms in bulk Pd. (e) Partial density of states projected on Pd atoms in a two-atomic-layer-thick Fe50Pd50alloy film on Pd(001). (f) The total density of states of a two-atomic-layer-thick Fe50Pd50alloy film on Pd(001). Figure 2: The magnon lifetime and spin-resolved density of states. ( a ) The magnon lifetime as a function of the wave vector. Solid squares represent the measured magnon lifetime of a two-atomic-layer-thick FePd alloy film on Pd(001) at T =13 K. The open squares and circles denote the calculated magnon lifetime for a two-atomic-layer-thick Fe 50 Pd 50 alloy film on Pd(001) and one atomic layer of Fe film on Pd(001), respectively. ( b ) The experimental magnon lifetime of the FePd alloy film (solid squares) compared with the one of a two-atomic-layer-thick Fe film on W(110) (empty circles). ( c ) The magnon linewidth as a function of the magnon energy. The results of the FePd alloy film on Pd(001) (solid circles) are compared with the ones of one atomic layer of Fe on W(110) (empty squares) and two atomic layers of Fe on W(110) (empty triangles). The dashed lines represent linear fits to the experimental data. ( d ) Density of states (DOS) of Pd atoms in bulk Pd. ( e ) Partial density of states projected on Pd atoms in a two-atomic-layer-thick Fe 50 Pd 50 alloy film on Pd(001). ( f ) The total density of states of a two-atomic-layer-thick Fe 50 Pd 50 alloy film on Pd(001). Full size image Magnetic exchange parameters We first attempt to shed light on the physics of magnetic excitations in this material by explaining the observed magnon dispersion relation. For that, we performed first-principles magnon calculations on the basis of ab initio density functional theory. To account for the alloy properties, we used a numerical scheme based on the coherent potential approximation (CPA) [33] , [34] , [35] , [36] . The strength of this scheme is that it properly takes into account the chemical disorder in the system. The electronic structure and magnetic properties are calculated using a self-consistent Green's function method and the magnetic exchange parameters are calculated using the magnetic force theorem approach again implemented within the Green function framework. The results of the calculations for a two-atomic-layer-thick Fe 50 Pd 50 random alloy film on Pd(001) are presented in Fig. 1c by the blue solid line. For comparison, we also present the results of the calculations for one-monolayer Fe film on Pd(001) (green solid line). The magnon mode shown in Fig. 1c satisfies the Goldstone theorem for which ε ( q =0)=0. The energy of terahertz magnons is determined by the interatomic magnetic exchange interaction. For the case of the Fe monolayer, the exchange interaction is confined to the plane of the monolayer. When Fe and Pd are interchanged forming a two-atomic-layer-thick alloy, the interaction between the atoms of different layers also becomes important. The pattern as well as the values of the exchange parameters change, and hence the dispersion relation for the two-atomic-layer-thick Fe 50 Pd 50 alloy film should be different from the one of the Fe monolayer. The analysis of the calculated magnetic exchange parameters reveals that the value of the Fe–Fe intralayer interaction (interaction in the same atomic plane) in the layer next to the Pd substrate is close to that of the Fe monolayer. The Fe–Fe interlayer interaction (interaction between atomic layers) is stronger than the intralayer exchange interaction (see Supplementary Table 1 and Supplementary Note 2 ). As a consequence, the magnon energies in the alloy film are higher than the ones in the Fe monolayer, in particular, for large wave vectors. The difference between the theoretical dispersion relation obtained for the two limiting cases is sizable for the direction and is small for the direction. The experimental values lie between two theoretical curves along the direction and just below both the theoretical curves along the direction. Since the prepared film is neither a perfect Fe monolayer nor a completely random Fe–Pd alloy, the overall agreement between experiment and theory can be considered as very good. Tailoring magnons’ energy The main contribution to the magnon dispersion relation comes from the Fe–Fe exchange parameters, since they are significantly larger than the Fe–Pd and Pd–Pd exchange parameters (see Supplementary Table 1 and Supplementary Note 2 ). It is apparent that a change in the Fe content would change the effective interatomic distances between Fe atoms and consequently would change the effective interatomic exchange interaction. This fact opens a possibility to tune the magnon energies (frequencies) by changing the Fe content. To realize this idea, we prepared a series of samples with different Fe content. The results of those experiments are summarized in Supplementary Note 3 and Supplementary Figure 2 . As the Fe content decreases the magnon energies decrease, demonstrating the possibility of tuning the magnon energies by changing the Fe content. Our next step is to understand the physics of the long magnons’ lifetime in this system with the aid of first-principles calculations within the framework of linear-response time-dependent density functional theory [12] . These calculations account properly for the magnons’ lifetime as they consider, on an equal footing, the collective magnetic excitations and single-particle Stoner excitations. The calculations are performed for two systems: one atomic layer of Fe film on the Pd(001) surface, and a two-atomic-layer-thick ordered Fe 50 Pd 50 supercell, mimicking the alloy film on Pd(001). The transverse dynamical spin susceptibility calculated using this scheme can be directly compared with the measured difference spectra. As in the experiment, the peak position denotes the energy and the linewidth indicates the lifetime of excitation. The calculated linewidth as a function of the wave vector is plotted in Fig. 1d and is compared with the one measured in the experiment. The agreement between theory and experiment is very good. We would like to emphasize that the observed long lifetime in the FePd system originates from the lower damping in this system, compared with other metallic ferromagnets. This may not be obvious from the linewidth versus wave vector data presented in Fig. 1d . In Fig. 2c , we plot the linewidth versus energy for the FePd system. The data are compared with the results of one and two atomic layers of Fe grown on W(110). At a given energy, the linewidth of excitations in the FePd system is smaller than that in the other systems. The energy dependence of the linewidth may be regarded as linear. Fitting the experimental data using a linear function provides a way of estimating the damping parameter, defined as Δ ε / ε . We find that the damping parameter in the FePd system is ~0.3 whereas in one-monolayer Fe/W(110) and two-monolayer Fe/W(110) is ~1.0 and 0.7, respectively. Obviously, the damping parameter in the FePd system is smaller than that in the Fe/W(110) system. The energy dependence of the linewidth in the FePd system is very similar to the one in the materials which are expected to exhibit a low damping, for example, yttrium iron garnet [19] and La 0.7 Ca 0.3 MnO 3 (a representative of magnetic oxides with half-metallic character) [37] . A comparison among different systems is provided in Supplementary Note 4 . As mentioned above, in itinerant ferromagnets, the Landau damping is the main mechanism governing the lifetime of terahertz magnons. Other processes like phonon and impurity scattering, multi-magnon scattering and spin–orbit damping may also be operative. However, they are much weaker than the Landau damping and hence are of second order importance. If one succeeds to engineer the electronic structure such that no (or very few) Stoner excitations are available near the Fermi level, one would suppress the Landau damping of magnons. If the density of states (DOS) of the material is modified such that the majority spin states are moved downwards or the minority spin states are moved upwards, one can suppress the low-energy Stoner excitations and thereby suppress the Landau damping of magnons. In principle, this can be done by a proper choice of materials combination. Figure 2d shows the density of states (DOS) of Pd atoms in paramagnetic Pd bulk. As it is apparent, the density of majority and minority electrons are identical, and, near the Fermi level, both majority and minority spin states exist. The total spin polarization is zero as it is expected for the Pd bulk. In addition, the Pd DOS features a characteristic peak just below the Fermi level. Figure 2e shows the partial DOS projected onto Pd atoms in a two-atomic-layer-thick Fe 50 Pd 50 alloy film. As it is apparent from Fig. 2e , when the Pd atoms are in the neighbourhood of Fe atoms, due to the strong hybridization of the electronic states, they become spin-polarized, which means that the majority states shift to lower energies leaving very little states near the Fermi level. This fact is also reflected in the total DOS of the Fe 50 Pd 50 alloy film, shown in Fig. 2f . The calculated DOS shown in Fig. 2d–f is consistent with the available experimental and theoretical results of the electronic structure of Pd/Fe(001) and Fe/Pd(001) (refs 38 , 39 ). The spin-polarizability of Pd atoms in the neighbourhood of Fe atoms is the key point explaining this phenomenon. Very low number of states near the Fermi level hinders the possibility of creation of Stoner excitations across the Fermi level leading to the long magnon lifetime. Exactly, the same phenomenon is expected when a monolayer of Fe is grown on the Pd(001) surface, as verified by our calculations. In literature, it is discussed that when a ferromagnet is in contact with a nonmagnetic metal, the hybridization of the electronic states of these two materials leads to an additional damping channel, decreasing the magnons’ lifetime in the ferromagnet [5] , [17] . This is based on the argument that the large density of states of the nonmagnetic metal near the Fermi level remain also in the total DOS of the whole system (ferromagnet plus nonmagnetic metal) leading to an additional possibility of creation of Stoner excitations. Our results demonstrate that this argument is not always true. A detailed knowledge of the electronic hybridization between the ferromagnet and nonmagnetic metal is essential to draw a conclusion about the damping. The lifetime depends on the wave vector and hence on the energy. To understand the energy and wave vector dependence of the lifetime, one should carefully investigate the spin- and momentum-resolved electronic bands, which contribute to the Landau damping of a magnon with given wave vector q and energy ε = ħω q ( ω denotes the eigenfrequency). For a magnon with a certain q and ε , one should consider all possible electron transitions from the majority bands to minority bands which create a single-particle electron–hole pair across the Fermi level with the momentum q and energy ε . To simply count the number of such transitions, one can rigidly shift the majority band by q and compare the majority states with momentum k ↑ − q and energy ε k ↑ − q ( k represents the electrons’ wave vector) with the minority states with momentum k ↓ and energy ε k ↓ for which the energy difference is . This follows the definition of a single-particle Stoner excitation with momentum q and energy ε , which is: one electron transition from an occupied majority state of k ↑ − q to minority state of k ↓ for which . 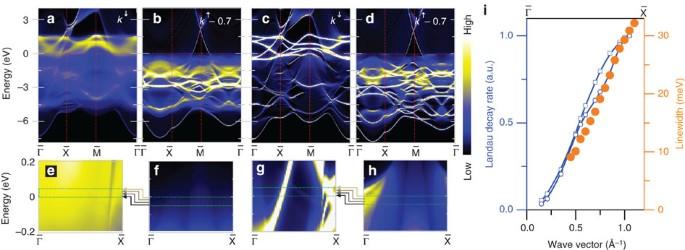Figure 3: The electronic bands and the Landau decay rate. (a–b) The spin- and momentum-resolved electronic bands of a two-atomic-layer-thick Fe50Pd50alloy film on Pd(001). (c–d) The spin- and momentum-resolved electronic bands of the Fe monolayer on Pd(001). (a,c) The minority states with momentumk↓. (b,d) The majority states with momentumk↑−q. The data are shown forq=0.7 Å−1. (e–h) The magnified parts ofa–dfor the small energies near the Fermi level. Possible Stoner transitions are schematically represented by the broken arrows. The colour bar represents the amplitude of the Bloch spectral function. The maximum and minimum amplitudes are represented by the white and black colours, respectively. (i) The Landau decay rate in the Fe50Pd50alloy film (open squares) and in the Fe monolayer (open circles) on Pd(001) versus wave vector. The right vertical axis shows the experimental magnon linewidth (solid circles) versus wave vector. Figure 3a,b show the spin and momentum resolved Bloch spectral functions of a two-atomic-layer-thick Fe 50 Pd 50 alloy film on Pd(001) calculated with the CPA approach. The minority states with momentum k ↓ are shown in a and the majority states with momentum k ↑ − q are shown in b . The same data for the Fe monolayer on Pd(001) are shown in Fig. 3c,d . The minority states with momentum k ↓ are shown in c and the majority states with momentum k ↑ − q are shown in d . In both cases, the Bloch spectral functions are projected into the two topmost atomic layers. As an example, we consider the case of q =0.7 Å −1 . The smearing of the bands shown in Fig. 3a,b is natural for a random alloy and is caused by disorder. Due to the fact that the majority bands are far from the Fermi level, this smearing has no influence on the analysis of the wave vector-dependent magnon damping. Since the magnon energies are in the range of 0 up to 120 meV, the interesting part of the electronic structure lies in the vicinity of the Fermi level (between ±120 meV), as only this part can contribute to the Landau damping of magnons. In Fig. 3e–h , the states close to the Fermi level are magnified. Figure 3e–h correspond to Fig. 3a–d , respectively. The Stoner transitions are schematically represented by the broken arrows. Figures 3e–h clearly indicate that near the Fermi level, only few majority states exist, which means that the possibility of creation of Stoner pairs is very low. As a result, the damping of magnons in this material is rather weak. To quantify the wave vector- and energy-dependent damping, we introduce the Landau decay rate, which describes the probability and the number of the possible decay channels of a magnon with a given q and ε to the Stoner excitations with the same q and ε . For q =0.7 Å −1 , the magnon energy is about ε =55 meV and hence the Stoner transitions from the region of −55 to +55 meV should be counted, since these transitions lead to the Landau damping of this particular magnon. The probability of an electron transition from an occupied majority state with momentum k ↑ − q to a minority state with momentum k ↓ is determined by the joint probabilities of finding an occupied state in k ↑ − q bands (initial state, ) and an empty state in k ↓ bands (final state, ). The total Landau decay rate will then be given by the following expression: , where ε f is the Fermi energy and P ( k ↑ − q , ε ) and P ( k ↓ , ε ) are the amplitudes of the Bloch spectral functions at the given k and ε , presented by the colour scale in Fig. 3a–h . Please note that the energy integral covers all the Stoner transitions in the energy region of ε f ± ε ( q ). The integration over k should be done over the surface Brillouin zone Ω BZ . Comparing Fig. 3a,b (or Fig. 3c,d ) reveals that the probability of Stoner transitions is mainly governed by the number of majority spin states, as there is an abundance of minority states available above the Fermi level. The Landau decay rate P ( q , ε ) can be calculated for each q and ε . Obviously, for a larger q , the energy ε is also larger and the integration over energy should be done over a larger energy range. Hence the number of Stoner transitions and consequently the Landau decay rate is larger. In Fig. 3i , the Landau decay rate, obtained by this method, is plotted versus q for the two-atomic-layer-thick Fe 50 Pd 50 film on Pd(001) and for the Fe monolayer on Pd(001). To be able to compare the results of these two systems, the values of each system are normalized to their maximum value at q =1.15 Å −1 . The experimental wave vector dependence of magnons’ linewidth is also plotted for a comparison. The increase of the Landau decay rate with increasing wave vector explains the wave vector (or energy)-dependent linewidth. Figure 3: The electronic bands and the Landau decay rate. ( a – b ) The spin- and momentum-resolved electronic bands of a two-atomic-layer-thick Fe 50 Pd 50 alloy film on Pd(001). ( c – d ) The spin- and momentum-resolved electronic bands of the Fe monolayer on Pd(001). ( a , c ) The minority states with momentum k ↓ . ( b , d ) The majority states with momentum k ↑ − q . The data are shown for q =0.7 Å −1 . ( e – h ) The magnified parts of a – d for the small energies near the Fermi level. Possible Stoner transitions are schematically represented by the broken arrows. The colour bar represents the amplitude of the Bloch spectral function. The maximum and minimum amplitudes are represented by the white and black colours, respectively. ( i ) The Landau decay rate in the Fe 50 Pd 50 alloy film (open squares) and in the Fe monolayer (open circles) on Pd(001) versus wave vector. The right vertical axis shows the experimental magnon linewidth (solid circles) versus wave vector. Full size image The Fe monolayer on Pd(001) has the same atomic structure as a two-atomic-layer-thick Fe 50 Pd 50 alloy film on Pd(001). The states of Fe atoms strongly hybridize with the states of the Pd atoms. Hence it is expected that the magnons in the Fe film shall possess properties similar to the ones in the alloy film. Another way of understanding the wave vector-dependent lifetime is to calculate the so-called Landau map and look for the Landau hot spots (the more the Landau hot spots, the larger the damping.) [11] , [12] . Two Landau maps are provided in Supplementary Fig. 3 for the Fe monolayer on Pd(001) at wave vectors of 0.2 and 0.7 Å −1 (For a detailed description of the Landau map, see Supplementary Note 5 and Supplementary Figure 3 ). The formation of the Landau hot spots can be traced back to the electronic structure. The position of the hot spots mark the places where the Stoner excitations are taking place with a large intensity. The Landau maps also indicate a weak damping of magnons in the Fe monolayer on Pd(001), as the number of hot spots is small and their intensity is low. 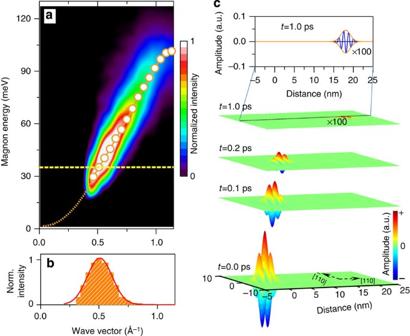Figure 4: Dynamics of the magnon wave packet. (a) The measured difference spectra plotted as a contour map. For a better representation, the values are normalized. The normalization is performed with respect to the maximum value. The open circles denote the position of the magnon peak. The dotted orange curve represents the extrapolation of the experimental data toq=0. The colour bar represents the normalized (norm.) intensity of the SPEELS difference spectra. (b) The distribution of magnon intensity in momentum space at the magnon energy ofε0=35 meV (along the dashed horizontal yellow line shown ina). It is well fitted by a Gaussian function as shown by the red solid curve. (c) Evolution of a magnon wave packet withε0=35 meV andq0=0.5 Å−1in real time and space. The images from bottom to top represent the wave packet in real space att=0, 0.1, 0.2 and 1.0 ps, respectively. The colour bar denotes the amplitude of the wave packet. The topmost graph shows a one-dimensional representation of the wave packet in real space att=1.0 ps. The amplitude of the wave packet at 1.0 ps is multiplied by 100 for clear visibility. After 1.0 ps, the wave packet has propagated around 18 nm. To visualize the dynamics of such long-lived magnons, we now use our experimental data to construct a magnon wave packet in real time and space (see Supplementary Note 6 and Supplementary Figure 4 for a detailed description of the procedure). The construction of the wave packet is based on the Fourier transformation of the magnon intensity from the momentum—energy space ( Fig. 4a ) to real position—time space. The reason that we construct the wave packet is to provide a clear picture of how a terahertz magnon wave packet propagates in this material. For information processing with terahertz magnons, one needs to know how fast the magnon wave packet moves, disperses and broadens in space while propagation. As an example, we show the magnon wave packet with the energy of ε 0 = ħω 0 =35 meV and the wave vector of q 0 =0.5 Å −1 , in the middle of the interval. In Fig. 4a , the dispersion relation is presented by open circles. The contour map represents the normalized intensity of the difference spectra (the normalization is performed with respect to the maximum value). The intensity distribution in the momentum space for the magnons with ε 0 =35 meV and q 0 =0.5 Å −1 is obtained directly by the line profile at ε 0 =35 meV (see Fig. 4a ). It can be well fitted by a Gaussian function represented by the red solid curve in Fig. 4b . Its full width at half maximum is ~0.2 Å −1 . A Fourier transformation results in the magnon wave packet in real space with a full width at half maximum of ~3 nm. The lifetime of the wave packet, defined as the time in which the amplitude of the wave packet is reduced by a factor of 1/ e , is about τ =130 femtoseconds (fs). The group velocity ε g = dω / dq , which can be obtained from the slope of the dispersion curve at ε 0 =35 meV and q 0 =0.5 Å −1 , is ~18 km s −1 . The evolution of the magnon wave packet in real time and space is shown in Fig. 4c . On the basis of the choice of scattering geometry, the magnons for which the momentum is parallel to the [110] direction at the surface of the film are excited. The wave packet starts to propagate at t =0, with the maximum amplitude at x =0. After t =1 ps, it propagates ~18 nm. During the propagation, the wave packet broadens in space very slowly. Its broadening in space is hardly visible in Fig. 4c . From application point of view, this can be regarded as an advantage. If the aim is to use this magnon wave packet for information transfer, one favours to have a wave packet which does not broaden in space very quickly. The animated movie of the propagation is shown in Supplementary Movie 1 . The lifetime of magnons in Fe films grown on W(110), at the wave vector of 0.5 Å −1 , is only 37 fs (refs 13 , 14 ). The amplitude of the wave packet reduces to 1% already after 0.17 ps. Its propagation length is only 4 nm. In the present case, the magnon wave packet survives for a longer time and propagates a longer distance. Figure 4: Dynamics of the magnon wave packet. ( a ) The measured difference spectra plotted as a contour map. For a better representation, the values are normalized. The normalization is performed with respect to the maximum value. The open circles denote the position of the magnon peak. The dotted orange curve represents the extrapolation of the experimental data to q =0. The colour bar represents the normalized (norm.) intensity of the SPEELS difference spectra. ( b ) The distribution of magnon intensity in momentum space at the magnon energy of ε 0 =35 meV (along the dashed horizontal yellow line shown in a ). It is well fitted by a Gaussian function as shown by the red solid curve. ( c ) Evolution of a magnon wave packet with ε 0 =35 meV and q 0 =0.5 Å −1 in real time and space. The images from bottom to top represent the wave packet in real space at t =0, 0.1, 0.2 and 1.0 ps, respectively. The colour bar denotes the amplitude of the wave packet. The topmost graph shows a one-dimensional representation of the wave packet in real space at t =1.0 ps. The amplitude of the wave packet at 1.0 ps is multiplied by 100 for clear visibility. After 1.0 ps, the wave packet has propagated around 18 nm. Full size image In summary, we report on the first observation of long-lived terahertz magnons excited in an ultrathin metallic alloy film (FePd). We shed light on the physical origin of the long lifetime of terahertz magnons in this compound, with the help of first-principles calculations. We show that the long magnon lifetime in this compound is due to the hybridization of the electronic states of Fe and Pd. In addition, we demonstrate that the magnon frequencies can be tuned by varying the Fe content. The long lifetime of magnons in this material, together with the possibility of tuning their excitation frequencies, make the compound an excellent candidate for terahertz magnonics. Since the FePd alloy is a good conductor, it can be simply integrated in the nowadays electronic devices. Experimental setup and sample preparation All experiments were carried out in an ultrahigh vacuum system (base pressure of 3 × 10 −11 mbar) equipped with Auger electron spectroscopy, low-energy electron diffraction, longitudinal magneto-optical Kerr effect (LMOKE) and SPEELS. Before the film deposition, the surface of Pd(001) single crystal was cleaned by cycles of Ar + sputtering at 1 keV until no contamination was detected by Auger electron spectroscopy and a subsequent annealing at 900 K. Clean Pd(001) surface shows a sharp 1 × 1 low-energy electron diffraction pattern. The films were deposited by an e-beam evaporator. The film thickness was calibrated by medium energy electron diffraction oscillations and cross-checked by the absolute value of Kerr ellipticity. After deposition, a mild annealing of the Fe monolayer on Pd(001) at 400 K for 10 min leads to a chemically disordered two-atomic-layer-thick face-centered tetragonal Fe 50 Pd 50 alloy film [21] . To avoid diffusion of Fe atoms into deeper Pd layers, we did not anneal the sample above 400 K. Here, we refer to an Fe coverage of one monolayer (atomic layer) as one adatom per substrate atom, that is, 1.32 × 10 15 atoms cm −2 . Magnetic characterization The magnetic state of the films was checked by LMOKE at 13 K. Our LMOKE experiments were carried out as a function of the temperature, the amount of Fe deposited on the surface and the direction of the external magnetic field. The magnetic field was applied along two main in-plane symmetry axes ([100] and directions). The results indicate that the hysteresis loop along both crystallographic directions is rectangular, meaning that both main symmetry axes show easy axis behaviour. The switching field at the measured temperature ( T =13 K) is about 25 Oe. The temperature dependence results provide an estimation of the Curie temperature of our films. For a two-atomic-layer FePd alloy film, it is ~370±10 K. The small magnetic anisotropy of the samples allowed us to saturate the magnetization of the film along any in-plane direction. SPEELS measurements The magnons were probed along a direction perpendicular to the magnetization. The sample was magnetized at 13 K before the SPEELS measurements and the spectra were recorded in the magnetic remanent state. To obtain a good signal-to-noise ratio, SPEELS measurements were performed at 13 K. A schematic representation of the scattering geometry is given in Fig. 1a . In the experiment, the incident electron energy was 6 eV and the degree of spin polarization of incident electrons was (72±5)%. The wave vector q of magnons is given by the scattering geometry: q = k i sin θ − k f sin ( θ 0 − θ ), where k i ( k f ) is the magnitude of the wave vector of the incident (scattered) electrons, and θ ( θ 0 ) is the angle between the incident beam and sample normal (the scattered beam). The momentum resolution is obtained by , here Δ θ =2°. It is ~0.03 Å −1 in our experiment [22] . Different wave vectors were achieved by changing the scattering angles. In our experiments, we fix the angle θ 0 on 80° and change θ by rotating the sample. First-principles calculations Three sets of calculations were performed. The first set of calculations was performed for the Fe monolayer on Pd(001) with structural parameters taken from the available experimental data [21] . The structural information served as the input for self-consistent calculations of the electronic structure within the framework of a generalized gradient approximation of density functional theory [40] . We adopted the Korringa–Kohn–Rostoker Green's function method and specially designed it for layered semi-infinite systems. The Heisenberg exchange constants were obtained by using the magnetic force theorem, implemented within the Green function method [41] . A second set of calculations was performed using a similar approach. To properly account for the alloy properties, a novel numerical scheme based on the coherent potential approximation (CPA) was used [33] , [34] , [35] , [36] . These calculations are performed for the case of Fe 50 Pd 50 alloy films. A third set of calculations was performed on the basis of linear-response time-dependent density functional theory [12] . This type of calculations provide information on the magnon lifetime in addition to the dispersion relation. How to cite this article: Qin, H. J. et al . Long-living terahertz magnons in ultrathin metallic ferromagnets. Nat. Commun. 6:6126 doi: 10.1038/ncomms7126 (2015).